Restoration of the third law in spin ice thin films A characteristic feature of spin ice is its apparent violation of the third law of thermodynamics. This leads to a number of interesting properties including the emergence of an effective vacuum for magnetic monopoles and their currents – magnetricity. Here we add a new dimension to the experimental study of spin ice by fabricating thin epitaxial films of Dy 2 Ti 2 O 7 , varying between 5 and 60 monolayers on an inert substrate. The films show the distinctive characteristics of spin ice at temperatures >2 K, but at lower temperature we find evidence of a zero entropy state. This restoration of the third law in spin ice thin films is consistent with a predicted strain-induced ordering of a very unusual type, previously discussed for analogous electrical systems. Our results show how the physics of frustrated pyrochlore magnets such as spin ice may be significantly modified in thin-film samples. Spin ice [1] illustrates much novel science, including unusual phases, degeneracies, quasiparticles and topology [1] , [2] , [3] , [4] , [5] , [6] , [7] , [8] , [9] . Its offshoots include artificial spin ice [10] , [11] and quantum spin ice [12] , [13] , while connections have been made with the physics of water ice [6] , electrolytes [14] , [15] , plasmas [16] and polariton condensates [17] . The canonical spin ice materials are the insulating oxides Ho 2 Ti 2 O 7 and Dy 2 Ti 2 O 7 , in which magnetic Ho 3+ or Dy 3+ occupy a pyrochlore lattice of linked tetrahedra [1] . The atomic magnetic moments or ‘spins’ of the rare earth ions map onto proton displacement vectors in water ice, so much of the rich physics of water ice, a strongly correlated proton system, is reproduced – remarkably – in these magnetic systems. Thus, local spin arrangements are controlled by an ‘ice rule’ that does not lead to long range order but instead stabilizes a correlated, disordered state with the Pauling ice entropy, S = R ln(3/2) per formula unit [2] . Microscopic modelling of spin ice [3] , [18] , [19] has suggested that, at sufficiently low temperature, the spin ice state becomes metastable with respect to an ordered ground state. For Dy 2 Ti 2 O 7 , a first estimate [18] put the ordering transition at 0.2 K, while a later estimate [19] , based on the fitting of neutron scattering data [20] , revised this estimate to <0.05 K. Direct evidence of the metastability was revealed in a recent and elegant calorimetric study [21] , which showed that on timescales of the order of a week, the residual entropy reduces to about 80% of the Pauling value at T =0.4 K, with a tendency to further reduction at lower temperature. It should be emphasized that the ‘frozen’ nature of the spin ice state is a consequence of the model of emergent magnetic monopoles [22] . Spin ice therefore represents an example where an apparent third law violation may be understood in detail in terms of quasiparticle dynamics (for the meaning of the third law in such metastable systems, see refs. 23 , 24 , and in the context of spin ice, the discussion in ref. 25 ). It nevertheless remains of particular interest to explore how the third law can be restored in spin ice. In this context, note that the well-established removal of spin ice entropy by an applied magnetic field [2] , [26] does not restore the third law but instead is a signal of its violation. The reason is that the third law requires the T =0 isotherm to be an isentrope [27] , so the entropy should be field independent. In contrast, lattice distortion gives a route to removing the spin ice entropy and unambiguously restoring the Third Law. Theory has predicted that a tetragonal distortion of cubic spin ice will lead to restoration of the third law in a thermodynamic transition of infinite order, of the type originally considered by Slater for the ferroelectric KDP [28] . However, the direct application of uniaxial pressure does not show clear evidence of this transition [29] , [30] , and one may conclude that the residual entropy of spin ice is robust against intrinsic ordering perturbations. The possibility of exploiting the unique magnetic properties of spin ice in devices motivated our study of spin ice in thin film form. Here we describe the fabrication of spin ice thin films and the characterization of their equilibrium thermodynamic properties. We fabricated the first single crystal epitaxial films of spin ice (here Dy 2 Ti 2 O 7 ) ranging from 5–60 nm thickness (Methods). For the substrate, we chose nominally diamagnetic Y 2 Ti 2 O 7 which is isostructural to Dy 2 Ti 2 O 7 , both being cubic pyrochlores, space group , cell constant a =1.0083, 1.0136, nm, respectively. The substrates were prepared as described in Methods and cut with edges defined by the crystallographic and [001] directions, and the normal to the plane defined by [110] (schematic in Fig. 1c ). The [110] surface was exposed to pulsed laser deposition of Dy 2 Ti 2 O 7 (Methods). Samples presented in this work will be referred as x DTO ∥ YTO(110), where x represents the total thickness of the Dy 2 Ti 2 O 7 layer in nanometres (note that 1 nm≈1 monolayer). Atomic force microscopy showed all films to be flat and smooth, with little or no evidence of terraces ( Supplementary Note 1 and Supplementary Figs 1–5 ). 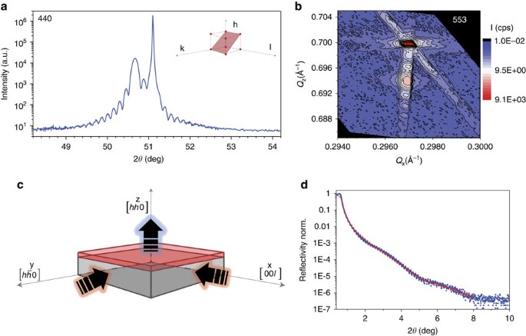Figure 1: The first spin ice films. Structural properties of Dy2Ti2O7∥Y2Ti2O7(110) at room temperature. (a) High-resolution XRD 2θ−ωscan of 60DTO∥YTO(110) (blue) showing (440) reflection for which we find out-of-plane lattice parameter ofa=1.018(1) nm for the film anda=1.011(1) nm for the substrate (Methods). Estimated thickness (Methods) is 60 nm. The inset shows the orientation of the (110) plane with respect to the crystallographic axes. (b) High-resolution XRD reciprocal space mapping showing (553) reflections of 60DTO∥YTO(110). Here,QxandQzare the components of the reciprocal space vector along the [00l] and [hh0] directions, respectively. The position of the weaker spot (film) near to the intense spot (substrate) shows the film to be epitaxial, but their coincidence inQxshows it to be fully strained along the [00l] direction (Methods). (c) Schematics of the actual orientation of the substrate (grey) and thin layer (red) with respect to the external reference systemxyz, along with the crystallographic orientations. Arrows indicates that the film appears to be stressed within the planexybut it is relaxed alongzinducing a distortion of the cubic symmetry. (d) Reflectivity measurement on 60DTO∥YTO(110) (blue). The red line is a fit, consistent with a film thickness of 62 nm, plus the presence of two thin interfaces at the top and at the bottom of the main layer (details in Methods). Figure 1: The first spin ice films. Structural properties of Dy 2 Ti 2 O 7 ∥ Y 2 Ti 2 O 7 (110) at room temperature. ( a ) High-resolution XRD 2 θ − ω scan of 60DTO ∥ YTO(110) (blue) showing (440) reflection for which we find out-of-plane lattice parameter of a =1.018(1) nm for the film and a =1.011(1) nm for the substrate (Methods). Estimated thickness (Methods) is 60 nm. The inset shows the orientation of the (110) plane with respect to the crystallographic axes. ( b ) High-resolution XRD reciprocal space mapping showing (553) reflections of 60DTO ∥ YTO(110). Here, Q x and Q z are the components of the reciprocal space vector along the [00 l ] and [ hh 0] directions, respectively. The position of the weaker spot (film) near to the intense spot (substrate) shows the film to be epitaxial, but their coincidence in Q x shows it to be fully strained along the [00 l ] direction (Methods). ( c ) Schematics of the actual orientation of the substrate (grey) and thin layer (red) with respect to the external reference system xyz , along with the crystallographic orientations. Arrows indicates that the film appears to be stressed within the plane xy but it is relaxed along z inducing a distortion of the cubic symmetry. ( d ) Reflectivity measurement on 60DTO ∥ YTO(110) (blue). The red line is a fit, consistent with a film thickness of 62 nm, plus the presence of two thin interfaces at the top and at the bottom of the main layer (details in Methods). Full size image Structural characterization of Dy 2 Ti 2 O 7 ∥ Y 2 Ti 2 O 7 The films were characterized by X-ray diffraction (XRD) to determine the orientation, epitaxy and thickness (Methods). The XRD pattern of room-temperature 60DTO ∥ YTO(110) is displayed in Fig. 1a ; the other scans are reported in Methods. The thickness of each sample was determined from the presence of fringes in the XRD pattern, as well as by fitting reflectivity curves. An example of a reflectivity measurement is reported in Fig. 1d (detailed analysis in Methods). The off-specular 553 reflection has been checked for all samples to confirm the epitaxial growth (data not reported here) and corroborate the crystal lattice constant (Methods). A reciprocal space map of the thickest sample ( Fig. 1b ) shows that the film is epitaxial and fully strained within the plane (Methods for more details). The stress induced by the substrate breaks the cubic symmetry of the thin layer and reduces the symmetry to tetragonal, or possibly lower. The departure from cubic symmetry of the films is sufficiently small (~0.8%, Methods), such that the distortion may be considered as a perturbation of the ideal spin ice system. Spin ice signatures Bulk spin ice exhibits three clear experimental signatures. First, the magnetic moment I saturates to different values along different crystallographic directions [31] , [32] , values that are both unusually large and particularly characteristic of spin ice. Second, the bulk isothermal susceptibility χ, when accurately corrected for demagnetization, displays an unusual departure from the Curie Law χ= C / T as a function of temperature [9] , [33] . Third, the magnetic entropy in zero field S ( T ) rises with temperature from the Pauling entropy S (0)= R ln(3/2) to a high temperature value of S ( T >10 K)≈2 R ln(2) (all entropies per mol Dy 2 Ti 2 O 7 ) [2] . In the absence of neutron scattering measurements (for which our samples are too small), these three thermodynamic signatures, when observed together on a single phase, may be taken as a definite confirmation of spin ice behaviour. Hence our investigation of the spin ice thin films focussed on the accurate measurement of these three quantities. 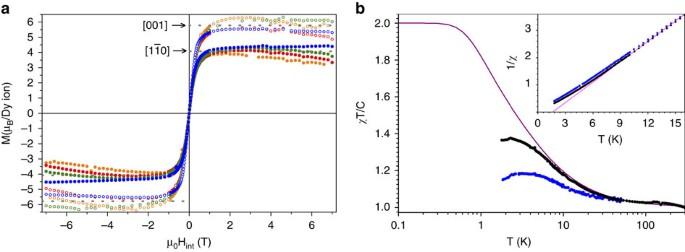Figure 2: Spin ice signatures. Magnetic properties of Dy2Ti2O7∥Y2Ti2O7. (a) Magnetization curves at 1.85 K along two principal axes [001] and. Colour code:xDTO∥YTO(110)x=60 (blue),x=40 (red),x=20 (green),x=5 (orange). Full and open circles correspond to the two orientations. Dashed lines show the expected saturated moments for the two-in, two-out spin configuration for each direction. (b) Temperature dependence of the dc susceptibility. Data are shown as the dimensionless quantity χT/Cversus temperature, from ref.33. Comparison between a bulk Dy2Ti2O7spherical crystal (black) and 60DTO∥YTO(110) (blue). The purple line is the calculated9,33quantity for Dy2Ti2O7. The inset shows the reciprocal susceptibility as a function of temperature for the same samples. The line is the best fit to an apparent Curie–Weiss lawχ=C′/(T−θ) with a Curie constantC′=4.25(5) K andθ=1.1(1) K. Magnetic moments Figure 2a summarizes measurements of the magnetic moment along [001] and , at T =1.85 K. These data have been corrected for a paramagnetic contribution arising from defects in Y 2 Ti 2 O 7 , estimated by direct measurement of the annealed substrate ( Supplementary Fig. 6 and Supplementary Note 2 ). Saturated moments along the [001] and directions agree with the expected values [31] , [32] for Ising spins constrained to the local 111 directions, shown as dashed lines in the figure. Deviations from the expected values may be due to a slight misalignment of the sample with respect to the applied field [32] as well as inaccuracies in background subtraction. Nevertheless, the correspondence between experiment and the expected saturation moment is striking, for the range of thickness explored here. Figure 2: Spin ice signatures. Magnetic properties of Dy 2 Ti 2 O 7 ∥ Y 2 Ti 2 O 7 . ( a ) Magnetization curves at 1.85 K along two principal axes [001] and . Colour code: x DTO ∥ YTO(110) x =60 (blue), x =40 (red), x =20 (green), x =5 (orange). Full and open circles correspond to the two orientations. Dashed lines show the expected saturated moments for the two-in, two-out spin configuration for each direction. ( b ) Temperature dependence of the dc susceptibility. Data are shown as the dimensionless quantity χ T / C versus temperature, from ref. 33 . Comparison between a bulk Dy 2 Ti 2 O 7 spherical crystal (black) and 60DTO ∥ YTO(110) (blue). The purple line is the calculated [9] , [33] quantity for Dy 2 Ti 2 O 7 . The inset shows the reciprocal susceptibility as a function of temperature for the same samples. The line is the best fit to an apparent Curie–Weiss law χ = C ′/( T − θ ) with a Curie constant C ′=4.25(5) K and θ =1.1(1) K. Full size image Curie Law crossover of Dy 2 Ti 2 O 7 ∥ Y 2 Ti 2 O 7 Figure 2b (inset) shows the measured reciprocal magnetic susceptibility of the thickest film, where it is seen to be close to that of the bulk, with the positive Curie–Weiss constant characteristic of spin ice, the frustrated ferromagnet ( Supplementary Fig. 7 shows χ( T ) for all samples). A more sensitive comparison with the bulk may be performed by plotting χ T / C as a function of temperature, as explained in ref. 33 (here C is the Curie constant). This test is shown in the main panel of Fig. 2b , where it is seen that the film behaves qualitatively like bulk spin ice, but that there are systematic deviations from the bulk behaviour, which become more significant at low temperature. Also shown in the figure is a model calculation for an expected ‘Curie Law Crossover’ [9] ( Fig. 2b ) that is observed in the bulk at high temperature [33] . The thin film data deviate from the model at a higher temperature than the data for bulk spin ice do. Bearing in mind the sensitivity of this analysis [33] , it is clear that the film behaves like a slightly perturbed spin ice at T >2 K. Magnetic entropy via specific heat To estimate the magnetic entropy, the measured heat capacity ( Fig. 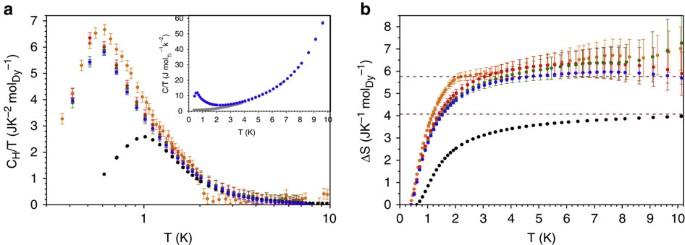Figure 3: Third law restoration in spin ice thin films. Magnetic specific heat and entropy increment of spin ice thin films and a comparison with bulk spin ice, Dy2Ti2O7. (a) Magnetic specific heat divided by temperature of a bulk crystal (black) and the films. Colour code:xDTO∥YTO(110)x=60 (blue),x=40 (red),x=20 (green),x=5 (orange). Error bars represent the estimated maximum systematic errors. The inset reports experimental data (before subtraction of the lattice contribution) related to the bare substrate (grey) and the thicker film plus substrate (blue) (Supplementary Note 3for more details). These data, showing the temperature dependence of the specific heat divided by temperatureC/Tper mole of Ti, clearly show a contribution below 4 K due to the presence of the thin spin ice layer. (b) Magnetic entropy increment found by integratingCH/Tbetween 0.35 K and 10 K for all the thin films and a bulk single crystal (same colour code is maintained in all figures). Error bars represent estimated maximum systematic error. Top dashed line corresponds to the expected value for the full spin entropy ofR(ln 2). The bottom dashed line corresponds to the expected value for a spin ice compound ofR(ln 2−(1/2) ln(3/2)), where the right hand term is the Pauling residual entropy. 3a and Supplementary Note 3 ) was corrected for the contribution of substrate and phonons and then integrated according to the following: Figure 3: Third law restoration in spin ice thin films. Magnetic specific heat and entropy increment of spin ice thin films and a comparison with bulk spin ice, Dy 2 Ti 2 O 7 . ( a ) Magnetic specific heat divided by temperature of a bulk crystal (black) and the films. Colour code: x DTO ∥ YTO(110) x =60 (blue), x =40 (red), x =20 (green), x =5 (orange). Error bars represent the estimated maximum systematic errors. The inset reports experimental data (before subtraction of the lattice contribution) related to the bare substrate (grey) and the thicker film plus substrate (blue) ( Supplementary Note 3 for more details). These data, showing the temperature dependence of the specific heat divided by temperature C / T per mole of Ti, clearly show a contribution below 4 K due to the presence of the thin spin ice layer. ( b ) Magnetic entropy increment found by integrating C H / T between 0.35 K and 10 K for all the thin films and a bulk single crystal (same colour code is maintained in all figures). Error bars represent estimated maximum systematic error. Top dashed line corresponds to the expected value for the full spin entropy of R (ln 2). The bottom dashed line corresponds to the expected value for a spin ice compound of R (ln 2−(1/2) ln(3/2)), where the right hand term is the Pauling residual entropy. Full size image where C H is the magnetic heat capacity at zero applied field. Setting , as in ref. 2 , the absolute entropy S ( T ) may be determined. As shown in Fig. 3a , significant differences between the heat capacity of the films and that of the bulk set in below T =2 K ( Fig. 3a ). For the films, this is reflected by a loss of all entropy by T 0 ≈0.3 , in contrast to the bulk, where the entropy saturates near Pauling’s value [2] . The fact that the entropy appears to approach zero at non-zero temperature suggests that the lowest energy excitations are gapped, as are emergent magnetic monopoles. Magnetic entropy via magnetization In order to check that all entropy is of a magnetic (electronic) origin, we determined the entropy by a different method, through the application of Maxwell’s relations to the measured magnetic moment I ( T , H ). This method, described in detail in ref. 34 , integrates the expression (∂ S /∂ H ) T = μ 0 (∂ I /∂ T ) H where μ 0 is the vacuum permeability. It gives accurate results for bulk spin ice and constitutes a robust independent test of the entropy of the thin spin ice films. It has the advantage over the calorimetric method of isolating the magnetic entropy on an absolute scale, without the complication of subtracting the lattice contribution [34] . The result is shown in Fig. 4 , where it is seen that a close agreement with the calorimetric result is achieved at T >2 K. Importantly, the observed value of the absolute entropy at 2 K ( Fig. 4 ) already indicates that any residual entropy in the films is much less than Pauling’s value. Having further excluded the possibility of systematic error in the calorimetry results at lower temperature ( Supplementary Note 3 , Supplementary Figs 8 and 9 ), we may conclude that magnetic entropy of the spin ice films tends to zero in accord with the Third Law. In contrast to bulk spin ice [2] , [21] , the zero entropy state of the thin films is achieved under laboratory conditions. The observed insensitivity of this result to film thickness shows that the entropy is an extensive property of the films and not related to their surfaces or boundaries. 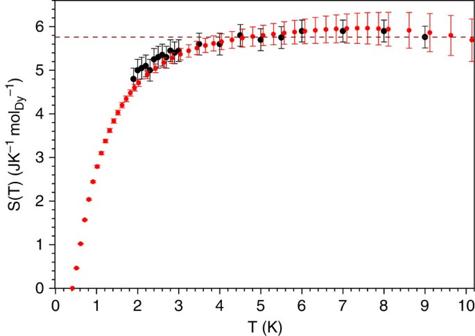Figure 4: Absolute determination of the magnetic entropy of Dy2Ti2O7∥Y2Ti2O7. Data correspond to the thickest sample 60DTO∥YTO(110). Comparison betweenS(T,Hint=0) derived by the magnetometry method34(black) with the entropy increment ΔS(T) derived by the calorimetric method (red). Error bars represent estimated maximum systematic error. Top dashed line corresponds to the expected value for the full spin entropy ofR(ln 2). Figure 4: Absolute determination of the magnetic entropy of Dy 2 Ti 2 O 7 ∥ Y 2 Ti 2 O 7 . Data correspond to the thickest sample 60DTO ∥ YTO(110). Comparison between S ( T , H int =0) derived by the magnetometry method [34] (black) with the entropy increment Δ S ( T ) derived by the calorimetric method (red). Error bars represent estimated maximum systematic error. Top dashed line corresponds to the expected value for the full spin entropy of R (ln 2). Full size image The conclusion from these experiments is clear: the films tend to typical spin ice behaviour at T >2 K and μ 0 H >1 T, but at lower temperature and zero field, they depart from spin ice behaviour. This is evidence of a new and relevant energy scale in the system. We consider the most likely origin of this energy scale is the strain in the films, which we estimate to be sufficient to remove the degeneracy. We derive a rough estimate of the strain by examining the difference in lattice constant between Dy 2 Ti 2 O 7 and Y 2 Ti 2 O 7 , which is of the same order of magnitude (though not necessarily of the same form) as that discussed in ref. 28 . We have considered ( Supplementary Note 4 ) the effect of this strain on the expected spin Hamiltonian of spin ice [3] , which is comprised of strongly strain-dependent exchange contributions and weakly strain-dependent dipolar contributions. A rough quantitative estimate (reported in Supplementary Note 4 ) suggests a consequent variation of the exchange interaction between 0.05 and 0.5 K, consistent with the onset of order and the observed loss of entropy in this temperature range. In the future, magnetic order could be tested directly by neutron scattering in larger samples, but it already seems likely that strain in the film plays a significant role in the loss of entropy. The situation appears to be analogous to the strain induced transition discussed in ref. 28 . Although we observe no clear evidence of a sharp transition in our specific heat data, we cannot rule out the possibility of a small specific heat peak that is either lost in the experimental noise or else at a temperature lower than those investigated. In conclusion, we have made the first thin films of Dy 2 Ti 2 O 7 spin ice. While this paper was under consideration, an independent group reported [35] thin films of Ho 2 Ti 2 O 7 spin ice with magnetization results consistent with our Fig. 2a . In our case, we have found that the degenerate spin ice state – which contains some microstates in a typical crystal – has finally yielded to the Third Law, plausibly as a result of strain induced by the lattice mismatch between film and substrate. We emphasize the comparison with bulk spin ice, where there is only a modest (20%) reduction of entropy by T ≈0.4 K and hence an insignificant loss of degeneracy [21] . In our films, the loss of entropy appears to be complete by this temperature. In the future it may be possible to modify the substrate to reduce strain and test for the possible recovery of the spin ice degeneracy. More generally, spin ice thin films facilitate the study of monopoles and magnetricity in an environment that is suited to direct space probes, and coupling to properties such as conduction electrons and electric fields [36] . Our result thus illustrates how the fabrication and study of thin films opens up new possibilities for the control and manipulation of the unusual magnetic properties of spin ice materials and related frustrated magnets. Choice of substrate, orientation and growth conditions In order to optimize growth conditions, several preliminary studies were conducted. One of the key parameters to obtain epitaxial films is the choice of the substrate: in particular, it is crucial to avoid the formation of multiple in-plane domains. Y 2 Ti 2 O 7 , which is iso-structural to Dy 2 Ti 2 O 7 and magnetically inert, is a logical choice, although it is not a conventional substrate for thin-film growth and it is not available commercially. Single crystals of Y 2 Ti 2 O 7 [37] were cut and epi-polished on one side (SurfaceNet GmbH, http://www.surfacenet.de ). A fully oriented set of substrates was obtained, for which one can customize the preferred orientations. In this paper, we report results for Dy 2 Ti 2 O 7 growth on Y 2 Ti 2 O 7 (110) where the in-plane edges were cut along (001) and , respectively. In a standard experiment, epitaxial films of Dy 2 Ti 2 O 7 were grown at 725 °C by pulsed laser deposition ( λ =248 nm, 8 cm target–substrate distance, fluence in the target 1.65 J cm −2 ) on one-side-polished 4 × 4 × 0.4 mm Y 2 Ti2O 7 (110) substrates that were fixed to a heater block with silver dag. Before growth, the substrates were annealed for 1 h at 750 °C after setting a 15 Pa flowing oxygen ambient. Growth temperature was adjusted ramping at 5 °C min −1 just before starting the deposition. Number of pulses were varied, according to Table 1 to obtain different film thickness. Samples were then annealed for 1 h setting a static 55 kPa oxygen pressure and reducing the temperature at 5 °C min −1 to 700 °C. Finally, the chamber was cooled to room temperature at 10 °C min −1 . Table 1 xDTO ∥ YTO(110): list of samples. Full size table Topography Film topography was studied with a VEECO Dimension 3100 Atomic Force Microscope (AFM) operated in tapping mode. Film surfaces were locally smooth, with a roughness of ~0.2–0.6 nm ( Supplementary Note 1 and Supplementary Figs 1–5 ). Structural characterization Lattice parameters and film epitaxy were studied by XRD using Cu K α1 radiation in a Rigaku high-resolution diffractometer. For each sample, the film thickness was determined from X-ray fringes. High-resolution reciprocal space maps of the thicker sample were collected using the same machine. Finally, reflectivity measurements were performed on two samples x DTO ∥ YTO(110) with x =60 and x =5. An out-of-plane orientation along the [110] direction has been confirmed for all the samples, as shown in Fig. 5 . From the presence of fringes, it is possible to estimate the thickness of each layer, as reported in Table 1 . For the thinnest sample, 5DTO ∥ YTO(110) ( Fig. 5d ), the thickness was estimated by comparison with the number of pulses used during the growth. 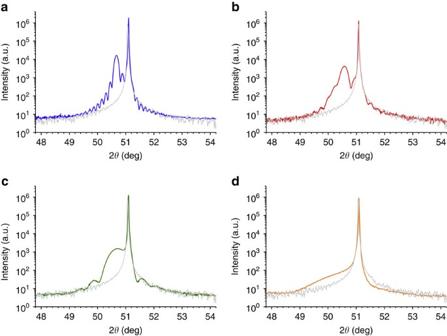Figure 5: Structural properties ofxDTO∥YTO(110) at room temperature. High-resolution XRD 2θ−ωscans. Annealed Y2Ti2O7substrate (grey) is plotted in all panels as reference and guide to the eye. We found a lattice parameter ofa=1.011(1) nm. (a)x=60 (blue) showing (440) reflection for which we found out-of-plane lattice parameter ofa=1.018(1) nm. Estimated thickness is 60 nm. (b)x=40 (red) showing (440) reflection for which we found out-of-plane lattice parameter ofa=1.018(1) nm. Estimated thickness is 40 nm. (c)x=20 (green) showing (440) reflection for which we find out-of-plane lattice parameter ofa=1.018(1) nm. Estimated thickness is 20 nm. (d)x=5 (orange) for which the (440) reflection is visible. No lattice parameter or thickness could be determined due to low intensity and broadness of the peak. Detailed analysis of all spectra is reported in Methods. Figure 5: Structural properties of x DTO ∥ YTO(110) at room temperature. High-resolution XRD 2 θ − ω scans. Annealed Y 2 Ti 2 O 7 substrate (grey) is plotted in all panels as reference and guide to the eye. We found a lattice parameter of a =1.011(1) nm. ( a ) x =60 (blue) showing (440) reflection for which we found out-of-plane lattice parameter of a =1.018(1) nm. Estimated thickness is 60 nm. ( b ) x =40 (red) showing (440) reflection for which we found out-of-plane lattice parameter of a =1.018(1) nm. Estimated thickness is 40 nm. ( c ) x =20 (green) showing (440) reflection for which we find out-of-plane lattice parameter of a =1.018(1) nm. Estimated thickness is 20 nm. ( d ) x =5 (orange) for which the (440) reflection is visible. No lattice parameter or thickness could be determined due to low intensity and broadness of the peak. Detailed analysis of all spectra is reported in Methods. Full size image For an independent estimate of the film thickness, two samples, x =60 and x =5, were characterized by X-ray reflectivity. 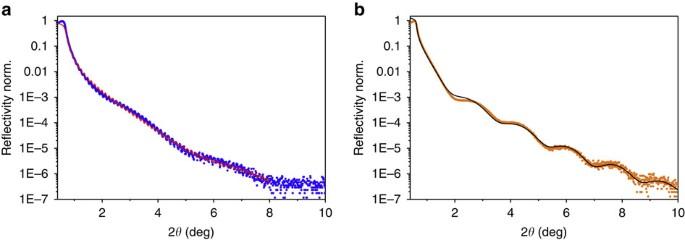Figure 6: Reflectivity ofxDTO∥YTO(110) at room temperature. Reflectivity measurement and related fit (solids lines –Supplementary Table S1) of (a)x=60 (blue). (b)x=5 (orange). Figure 6 reports the two reflectivity curves with related fits. The fits were performed with the Integrated Thin Film Analysis Software GlobalFit 1.3 (Rigaku Corporation). The background was not measured, but was included as a fitting parameter. The main purpose of this analysis was to extrapolate the thickness of the film and the density of the main layer, both of which are expected to be reliable numbers in our analysis. A simple analysis of the roughness was included but is likely to be less accurate than the film thickness; the roughness parameters are reported in Supplementary Table 1 just for completeness. The multilayer structure consists of the presence of a main layer with two interfaces, one at the bottom and one at the top of the film. The calculated total thicknesses are in good agreement with the nominal expected values. Furthermore, the density of the film is close to the tabulated bulk density of Dy 2 Ti 2 O 7 . Figure 6: Reflectivity of x DTO ∥ YTO(110) at room temperature. Reflectivity measurement and related fit (solids lines – Supplementary Table S1 ) of ( a ) x =60 (blue). ( b ) x =5 (orange). Full size image Referring to the reciprocal space mapping reported in Fig. 1b , it is possible to draw some conclusions. The relative positions of reciprocal lattice points of an epitaxial film and its substrate change, depending on lattice matching and the presence or absence of lattice distortion. 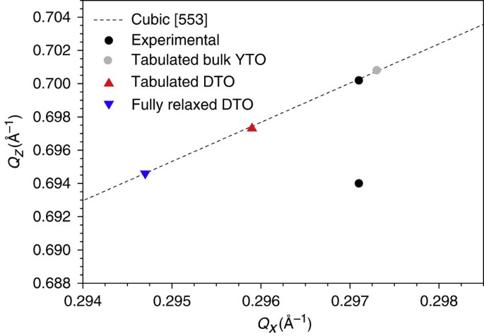Figure 7: Reciprocal space mapping of bulk and epitaxial films of spin ices. Here,QxandQzare the components of the reciprocal space vector along the [00l] and [hh0] directions, respectively. The plot shows the positions in reciprocal space of the (553) reciprocal lattice point for bulk Y2Ti2O7(grey dot) and Dy2Ti2O7(red triangle) based on tabulated lattice parameters38. Both lie along the line for the cubic lattice (dotted line). The experimental data (Fig. 1b) show how the substrate maintained the expected cubic structure (upper black dot), with only a very slightly different lattice constant. The Dy2Ti2O7film (lower black dot), however, is strained along the [00l] direction – see text for the details. For completeness, the reciprocal (553) reciprocal lattice point for a hypothetical fully relaxed film (blue inverted triangle) is shown, assuming the cubic structure but with lattice constant obtained from the symmetric (440) reflection (Fig. 5). Note that error bars are within the symbol size. Figure 7 schematically illustrates the reciprocal space maps for relaxed and strained films. Here we denote an epitaxial film having the same cubic crystal structure as the bulk with the same out of plane lattice constant as the real film, as a ‘fully relaxed’ state. For such a fully relaxed state, the unit cell would be uniformly expanded compared with the substrate, and so the reciprocal lattice point of the film with indices (553) would lie on the line connecting the reciprocal lattice point (553) of the substrate with the origin of reciprocal space (dotted line of Fig. 7 ). Our experimental data (black dots of Fig. 7 ) show that the (553) reciprocal lattice point of the film is not positioned on this line, but instead is positioned directly below (on Fig. 1b ) the (553) point of the substrate for both symmetric ( Fig. 5 ) and asymmetric diffraction. This suggests that the lattice of the film is strained in a manner such that the in-plane lattice constant of the epitaxial film and those of the substrate match, at least along the [00 l ] direction. Note that this is a very small (0.7–0.8%) strain which is not expected to significantly affect atomic positions in the nearly cubic unit cell. As well as being compressed within the plane of the film, the unit cell appears to be elongated along the out of plane direction. Hence, the hypothetical fully relaxed state has a slightly enlarged unit cell volume compared with the bulk, whereas the real films maintain approximately the same unit cell volume. Figure 7: Reciprocal space mapping of bulk and epitaxial films of spin ices. Here, Q x and Q z are the components of the reciprocal space vector along the [00 l ] and [ hh 0] directions, respectively. The plot shows the positions in reciprocal space of the (553) reciprocal lattice point for bulk Y 2 Ti 2 O 7 (grey dot) and Dy 2 Ti 2 O 7 (red triangle) based on tabulated lattice parameters [38] . Both lie along the line for the cubic lattice (dotted line). The experimental data ( Fig. 1b ) show how the substrate maintained the expected cubic structure (upper black dot), with only a very slightly different lattice constant. The Dy 2 Ti 2 O 7 film (lower black dot), however, is strained along the [00 l ] direction – see text for the details. For completeness, the reciprocal (553) reciprocal lattice point for a hypothetical fully relaxed film (blue inverted triangle) is shown, assuming the cubic structure but with lattice constant obtained from the symmetric (440) reflection ( Fig. 5 ). Note that error bars are within the symbol size. Full size image Crystal lattice constants of both substrate and film (reported in Fig. 5 ) were determined, as described below. Bulk Y 2 Ti 2 O 7 and Dy 2 Ti 2 O 7 tabulated [38] cubic constants are a =1.0083, nm and a =1.0136, nm, respectively. The substrates do not show any distortion and the lattice constant obtained from both (440) and (553) reflections is a =1.011(1) nm. Figure 5 and Fig. 1a show that the d 110 spacing of the Y 2 Ti 2 O 7 substrates are smaller than those of the thin layers of Dy 2 Ti 2 O 7 , in line with the expected bulk values. On the other hand, off-specular (553) reflections (pattern not shown, but see Fig. 1b for the thicker sample) suggest that the films are strained within the plane, at least along the [00 l ] direction. We have not yet characterized the third independent direction, , so it is not possible to identify the actual distortion, that is, tetragonal or monoclinic. Nevertheless, in order to have an estimate of the lattice constant, we considered the simplest case of a tetragonal distortion, where a = b ≠ c , for which we can solve the problem having measured the (440) and (553) reflections. The lattice constants obtained under such assumption are a = b =1.018(1) nm and c =1.011(1) nm. Magnetic properties In-plane magnetization was measured using a Quantum Design MPMS-7 SQUID (Superconducting Quantum Interference Device) magnetometer. Measurements were performed in RSO (Reciprocating Sample Option) operating mode to achieve better sensitivity by eliminating low-frequency noise. Silver dag was removed from the underside of samples to prevent the possibility of spurious magnetic signals attributed to material from the heater block in the deposition system. Samples were positioned using a customized sample-holder to avoid displacement or reorientation during the measurement. Finally the holder was loaded inside a clear plastic drinking straw, of 5 mm diameter. The arrangement of coils in the MPMS-7 ideally allows complete cancellation of background signals from the sample holder and strongly reduces the effect of field noise in the magnet. Specific heat The specific heat of each sample was measured in the temperature range between 0.35 K and 50 K with a Quantum Design PPMS (Physical Properties Measurement System) with a 3 He option. The data were corrected for the addenda heat capacity, which was measured in a separate run. Magnetic entropy via magnetization To estimate the magnetic entropy via magnetization, we followed the procedure described in ref. 34 . Experimentally, we measured the magnetization at different temperatures as a function of applied field on two different systems, a Quantum Design SQUID magnetometer ( μ 0 H max =7 T) and a vibrating sample magnetometer measurement system for the Quantum Design PPMS ( μ 0 H max =14 T). Magnetic fields were applied along the [001] axis – within the plane of the thin films. The magnetic moment I versus H applied was measured at many temperatures in the range 1.8≤ T /K≤10 (typically every 0.1 K). For details of the data analysis method, we refer to ref. 34 . How to cite this article: Bovo, L. et al. Restoration of the third law in spin ice thin films. Nat. Commun. 5:3439 doi: 10.1038/ncomms4439 (2014).